PI(3,5)P2controls membrane trafficking by direct activation of mucolipin Ca2+release channels in the endolysosome Membrane fusion and fission events in intracellular trafficking are controlled by both intraluminal Ca 2+ release and phosphoinositide (PIP) signalling. However, the molecular identities of the Ca 2+ release channels and the target proteins of PIPs are elusive. In this paper, by direct patch-clamping of the endolysosomal membrane, we report that PI(3,5)P 2 , an endolysosome-specific PIP, binds and activates endolysosome-localized mucolipin transient receptor potential (TRPML) channels with specificity and potency. Both PI(3,5)P 2 -deficient cells and cells that lack TRPML1 exhibited enlarged endolysosomes/vacuoles and trafficking defects in the late endocytic pathway. We find that the enlarged vacuole phenotype observed in PI(3,5)P 2 -deficient mouse fibroblasts is suppressed by overexpression of TRPML1. Notably, this PI(3,5)P 2 -dependent regulation of TRPML1 is evolutionarily conserved. In budding yeast, hyperosmotic stress induces Ca 2+ release from the vacuole. In this study, we show that this release requires both PI(3,5)P 2 production and a yeast functional TRPML homologue. We propose that TRPMLs regulate membrane trafficking by transducing information regarding PI(3,5)P 2 levels into changes in juxtaorganellar Ca 2+ , thereby triggering membrane fusion/fission events. Ca 2+ is a key regulator of synaptic vesicle fusion during neurotransmission. Similarly, Ca 2+ is thought to regulate other, more general membrane trafficking pathways [1] . However, in these cases, the source of Ca 2+ is unknown. For these general pathways, it has been postulated that Ca 2+ is released through unidentified Ca 2+ channels from the lumen of vesicles and organelles [1] , [2] , [3] . Transient receptor potential (TRP) proteins are members of a superfamily of Ca 2+ -permeable cation channels that are localized at the plasma membrane and/or membranes of intracellular organelles [4] . For example, mucolipin TRPs (TRPML1–3) are localized in the membranes of endosomes and lysosomes (collectively endolysosomes) [5] , [6] . Mutations in the human TRPML1 gene cause mucolipidosis type IV (ML4) neurodegenerative disease [7] , [8] . Cells that lack TRPML1 exhibit enlarged endolysosomes and trafficking defects in the late endocytic pathway (reviewed by Cheng et al . [5] and Puertollano and Kiselyov [6] ). TRPMLs are, therefore, natural candidate channels for Ca 2+ release in the endolysosome. PI(3,5)P 2 is a low-abundance endolysosome-specific phosphoinositide (PIP) [9] , [10] , [11] , [12] . PI(3,5)P 2 can be generated from PI(3)P through PIKfyve/Fab1, a PI 5 kinase that is localized in the endolysosome of both yeast and mammalian cells [11] , [13] , [14] , [15] . The activity of PIKfyve/Fab1 can be positively regulated by several associated proteins such as Fig4, Vac14 and Vac7 [10] , [11] , [12] , [16] . On the other hand, PI(3,5)P 2 can be metabolized into PI(5)P through the myotubularin (MTM/MTMR) family of PI 3 phosphatase [11] , [15] , [17] . Human mutations in PI(3,5)P 2 -metabolizing enzymes and their regulators cause various neurodegenerative diseases, including amyotrophic lateral sclerosis and Charcot-Marie-Tooth disease [10] , [11] , [18] . At the cellular level, PI(3,5)P 2 -deficient cells reportedly exhibit enlarged endolysosomes/vacuoles and trafficking defects in endocytic pathways [10] , [11] , [12] , [16] . Because the cellular phenotypes in PI(3,5)P 2 -deficient cells are similar to those observed in cells lacking TRPML1, we hypothesized that TRPML1 may function as an endolysosomal Ca 2+ release channel that is regulated by PI(3,5)P 2 . In this study, by direct patch-clamping of the endolysosomal membrane, we found that PI(3,5)P 2 activates TRPMLs with striking specificity and potency. Protein–lipid interaction and mutational analyses revealed that PI(3,5)P 2 binds directly to the N terminus of TRPML1. Overexpression of TRPML1 suppresses the enlarged vacuole phenotype observed in PI(3,5)P 2 -deficient cells. We conclude that PI(3,5)P 2 controls endolysosomal membrane trafficking by regulating TRPML channels to change juxtaorganellar Ca 2+ levels. Activation of endolysosomal TRPML channels by PI(3,5)P 2 TRPML1 is primarily localized on membranes of late endosomes and lysosomes (LELs) [5] , [19] (see Supplementary Fig. S1 ), which are inaccessible to conventional electrophysiological approaches. Using our recently established modified patch-clamp method [4] , [20] , we performed recordings directly on native LEL membranes. HEK293 T or Cos-1 cells were transfected with either enhanced green fluorescent protein (EGFP)-TRPML1 alone, or co-transfected with mCherry-TRPML1 and EGFP-Lamp1 (a marker for LEL). Whole-endolysosome recordings (see Fig. 1a ; note that the inward current indicates cations flowing out of the endolysosome) were performed on enlarged vacuoles manually isolated from cells pretreated with vacuolin-1 [21] , which caused an increase in the diameter of vacuoles from <0.5 μm to up to 5 μm (mean capacitance=0.68±0.05 pF, N =44 vacuoles). The majority (>85%) of mCherry-TRPML1-positive vacuoles were also EGFP-Lamp1 positive, confirming that TRPML1-positive vacuoles were enlarged LELs [21] . In TRPML1-positive enlarged LELs, small basal inwardly rectifying currents (72±12 pA/pF at −140 mV, N =65 vacuoles) were seen under the whole-endolysosome configuration ( Fig. 1b,c ). Bath application of 100 nM PI(3,5)P 2 in a water-soluble diC8 form rapidly and dramatically activated a TRPML1-mediated current ( I TRPML1 ; τ =15±4 s at −140 mV, N =8 vacuoles; 18.3±2.7-fold increase in basal activity, N =20 vacuoles) ( Fig. 1b–f ). PI(3,5)P 2 -dependent activation was dose dependent (EC 50 =48±14 nM, Hill slope ( n )=1.9, N =7 vacuoles). On average, I TRPML1 in the presence of 100 nM diC8 PI(3,5)P 2 was 982±150 pA/pF at −140 mV ( N =23 vacuoles). Full-length diC16 PI(3,5)P 2 seemed to be less effective, presumably because of its low aqueous solubility ( Supplementary Fig. S2 ). Therefore, diC8 PI(3,5)P 2 was used for electrophysiological studies hereafter. 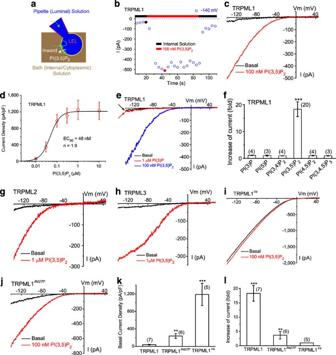Figure 1: PI(3,5)P2activates recombinant TRPML channels in the endolysosomal membranes. (a) Illustration of a whole-endolysosome recording configuration. Pipette (luminal) solution was a standard external (Tyrode's) solution adjusted to pH 4.6 to mimic the acidic environment of the lysosome lumen. Bath (internal/cytoplasmic) solution was a K+-based solution (140 mM K+-gluconate). Putative membrane topology of TRPML channels is illustrated in the late endosome and lysosome (LEL). Note that the inward current indicates cations flowing out of the endolysosome (see white arrow for the direction). (b) Bath application of PI(3,5)P2(diC8, 100 nM) activated inwardly rectifying whole-endolysosome TRPML1-mediated current (ITRPML1) in an enlarged endolysosome/vacuole from a TRPML1-EGFP-expressing Cos-1 cell that was pretreated with vacuolin-1.ITRPML1was elicited by repeated voltage ramps (−140 to +140 mV; 400 ms) with a 4-s interval between ramps.ITRPML1exhibited a small basal current before PI(3,5)P2application; bath application of PI(3,5)P2to the cytoplasmic side of the endolysosome resulted in maximal activation of 18-fold of baseline within a minute, measured at −140 mV ofITRPML1. (c) Representative traces ofITRPML1before (black) and after (red) PI(3,5)P2at two time points, as shown ina(black and red circles). Only a portion of the voltage protocol is shown; holding potential=0 mV. (d) Dose-dependence of PI(3,5)P2-dependent activation (EC50=48 nM,n=1.9). (e) PI(3)P (1 μM) failed to activateITRPML1. (f) Specific activation of TRPML1 by PI(3,5)P2(in 100 nM), but not other diC8 PIPs (all in 1 μM). (g) Activation of whole-endolysosomeITRPML2by PI(3,5)P2(1 μM). (h) Activation of whole-endolysosomeITRPML3by PI(3,5)P2(1 μM). (i) Whole-endolysosomeITRPML1-Vaexhibited high basal activity but was insensitive to PI(3,5)P2(100 nM). (j) Whole-endolysosomeITRPML1-R427Pwas weakly activated by PI(3,5)P2. (k) Basal current amplitudes of whole-endolysosomeITRPML1,ITRPML1-R427PandITRPML1-Va. (l) Effects of PI(3,5)P2onITRPML1,ITRPML1-R427PandITRPML1-Va. Ford,f,k,l, data are presented as the mean ± s.e.m.; thennumbers are in parentheses. Statistical comparisons were made using analysis of variance: **P<0.01; ***P<0.001. Figure 1: PI(3,5)P 2 activates recombinant TRPML channels in the endolysosomal membranes. ( a ) Illustration of a whole-endolysosome recording configuration. Pipette (luminal) solution was a standard external (Tyrode's) solution adjusted to pH 4.6 to mimic the acidic environment of the lysosome lumen. Bath (internal/cytoplasmic) solution was a K + -based solution (140 mM K + -gluconate). Putative membrane topology of TRPML channels is illustrated in the late endosome and lysosome (LEL). Note that the inward current indicates cations flowing out of the endolysosome (see white arrow for the direction). ( b ) Bath application of PI(3,5)P 2 (diC8, 100 nM) activated inwardly rectifying whole-endolysosome TRPML1-mediated current ( I TRPML1 ) in an enlarged endolysosome/vacuole from a TRPML1-EGFP-expressing Cos-1 cell that was pretreated with vacuolin-1. I TRPML1 was elicited by repeated voltage ramps (−140 to +140 mV; 400 ms) with a 4-s interval between ramps. I TRPML1 exhibited a small basal current before PI(3,5)P 2 application; bath application of PI(3,5)P 2 to the cytoplasmic side of the endolysosome resulted in maximal activation of 18-fold of baseline within a minute, measured at −140 mV of I TRPML1 . ( c ) Representative traces of I TRPML1 before (black) and after (red) PI(3,5)P 2 at two time points, as shown in a (black and red circles). Only a portion of the voltage protocol is shown; holding potential=0 mV. ( d ) Dose-dependence of PI(3,5)P 2 -dependent activation (EC 50 =48 nM, n =1.9). ( e ) PI(3)P (1 μM) failed to activate I TRPML1 . ( f ) Specific activation of TRPML1 by PI(3,5)P 2 (in 100 nM), but not other diC8 PIPs (all in 1 μM). ( g ) Activation of whole-endolysosome I TRPML2 by PI(3,5)P 2 (1 μM). ( h ) Activation of whole-endolysosome I TRPML3 by PI(3,5)P 2 (1 μM). ( i ) Whole-endolysosome I TRPML1-Va exhibited high basal activity but was insensitive to PI(3,5)P 2 (100 nM). ( j ) Whole-endolysosome I TRPML1-R427P was weakly activated by PI(3,5)P 2 . ( k ) Basal current amplitudes of whole-endolysosome I TRPML1 , I TRPML1-R427P and I TRPML1-Va . ( l ) Effects of PI(3,5)P 2 on I TRPML1 , I TRPML1-R427P and I TRPML1-Va . For d , f , k , l , data are presented as the mean ± s.e.m. ; the n numbers are in parentheses. Statistical comparisons were made using analysis of variance: ** P <0.01; *** P <0.001. Full size image In yeast, PI(3,5)P 2 is exclusively produced from PI(3)P by the PIKfyve/Fab1 PI 5 kinase (see Supplementary Fig. S1 ) [9] , [22] , [23] . PI(3,5)P 2 can be quickly metabolized into PI(3)P by Fig4, or to PI(5)P by the MTMR family of phosphatases [11] , [13] , [17] , [24] . Neither PI(3)P (1 μM; 1.05±0.17-fold increase in basal, N =4; Fig. 1e,f ) nor PI(5)P (1 μM; 0.98±0.05-fold increase in basal, N =3; Fig. 1f ) activated I TRPML1 . PI(3)P and PI(3,5)P 2 are localized in the endolysosome system. Other PIPs such as PI(3,4)P 2 , PI(4,5)P 2 and PI(3,4,5)P 3 are localized in the plasma membrane, or in other intracellular organelles, and are sequestered from endolysosomes [15] . I TRPML1 was not activated by these other PIPs ( Fig. 1f and Supplementary Fig. S3 ). Thus, PI(3,5)P 2 activated I TRPML1 with a striking specificity. TRPML2 and TRPML3 are also localized in the endolysosome [5] . PI(3,5)P 2 , but not PI(3)P (data not shown), activated whole-endolysosome I TRPML2 ( Fig. 1g ) and I TRPML3 ( Fig. 1h ). As PI(3,5)P 2 and TRPMLs are both primarily localized in the LEL [5] , [11] (see Supplementary Fig. S4 ), the insensitivity of I TRPML1 to PI(3)P or PI(5)P, and its robust activation by PI(3,5)P 2 , suggested that TRPML1 might be acutely regulated by the activities of PIKfyve/Fab1, or by Fig4 or MTMR phosphatases in the LEL. PI(3,5)P 2 -mediated activation gating of TRPML1 To explore the mechanisms underlying PI(3,5)P 2 -dependent activation of TRPMLs, we tested the effect of PI(3,5)P 2 on several gain-of-function mutations in TRPML1 channels [20] . Recently, we, along with others, found that a spontaneous mutation ( Varitint Waddler ; Va ) in the fifth transmembrane domain of TRPML3 dramatically increased TRPML3 channel activity [5] , [6] . Further analysis suggested that Va is a gating mutation that locks TRPML1-3 channels in an open non-gating state [5] , [6] . In contrast with I TRPML1 , whole-endolysosome I TRPML1-Va exhibited large basal currents (1,190±254 pA/pF at −140 mV, N =5) that failed to increase with PI(3,5)P 2 application (0.99±0.01 of basal, N =3; Fig. 1i,k,l ). TRPML1-R427P is a partial gain-of-function mutation [20] . Whole-endolysosome I TRPML1-R427P exhibited a substantial basal current (349±80 pA/pF at −140 mV, N =3), but was only modestly activated by PI(3,5)P 2 at 3.7±1.3-fold of basal activity ( N =7) ( Fig. 1j–l ). Collectively, these results suggested that PI(3,5)P 2 activated TRPML1 by increasing the open probability. Activation of endogenous TRPML-like currents by PI(3,5)P 2 Next, we investigated whether PI(3,5)P 2 activated endogenous TRPMLs. Using enlarged LELs isolated from non-transfected Cos-1 cells, we were able to record PI(3,5)P 2 -activated, inwardly rectifying TRPML-like currents ( I TRPML-L ) in 4 out of 20 vacuoles ( Fig. 2a ). I TRPML-L was 68±4 pA/pF at −140 mV ( N =4). In enlarged LELs isolated from wild-type (WT) (TRPML1 +/+ ) human fibroblast cells, however, PI(3,5)P 2 -activated I TRPML-L was detected in five of five tested vacuoles ( Fig. 2b ), with an average current amplitude larger than that of Cos-1 cells (239±37 pA/pF at −140 mV, N =5; Fig. 2d ). In contrast, enlarged LELs from human ML4 (TRPML1 −/− or abbreviated as ML1 −/− ) fibroblasts showed no significant PI(3,5)P 2 -activated I TRPML-L (15.7±5.2 pA/pF at −140 mV, N =6; Fig. 2c,d ). These results indicated that PI(3,5)P 2 activated endogenous TRPMLs, and that TRPML1 was the primary or sole functional TRPML channel in the endolysosome of human fibroblasts, although a previous study reported the expression of TRPML2 and TRPML3 in human fibroblasts [25] . 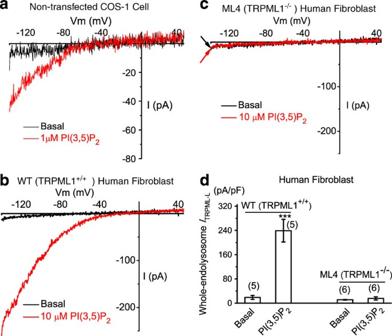Figure 2: PI(3,5)P2activates endogenous TRPML-like currents (ITRPML1-L) in the endolysosomal membranes. (a) An endogenous inwardly rectifyingITRPML1-Lactivated by PI(3,5)P2(10 μM) in a vacuole isolated from a non-transfected Cos-1 cell. (b) Large PI(3,5)P2-activatedITRPML1-Lin a vacuole isolated from wild-type (WT) human skin fibroblast cell. (c) Lack of significant PI(3,5)P2-activatedITRPML1-Lin a vacuole isolated from a human ML4 (TRPML1−/−) skin fibroblast cell. (d) Endogenous PI(3,5)P2-activatedITRPML-Lin WT and TRPML1−/−human fibroblasts. Data are presented as the mean ± s.e.m.; thennumbers are in parentheses. Statistical comparisons were made using analysis of variance: ***P<0.001. Figure 2: PI(3,5)P 2 activates endogenous TRPML-like currents ( I TRPML1-L ) in the endolysosomal membranes. ( a ) An endogenous inwardly rectifying I TRPML1-L activated by PI(3,5)P 2 (10 μM) in a vacuole isolated from a non-transfected Cos-1 cell. ( b ) Large PI(3,5)P 2 -activated I TRPML1-L in a vacuole isolated from wild-type (WT) human skin fibroblast cell. ( c ) Lack of significant PI(3,5)P 2 -activated I TRPML1-L in a vacuole isolated from a human ML4 (TRPML1 −/− ) skin fibroblast cell. ( d ) Endogenous PI(3,5)P 2 -activated I TRPML-L in WT and TRPML1 −/− human fibroblasts. Data are presented as the mean ± s.e.m. ; the n numbers are in parentheses. Statistical comparisons were made using analysis of variance: *** P <0.001. Full size image Suppression of I TRPML1 by a decrease in PI(3,5)P 2 Whole-endolysosome I TRPML1 exhibited a decay or slow return to steady-state levels on washout of diC8 PI(3,5)P 2 ( Fig. 3a ). If PI(3,5)P 2 levels underlie the basal pre-PI(3,5)P 2 , or the post-PI(3,5)P 2 activity of TRPML1, diminishing the PI(3,5)P 2 level would be expected to decrease I TRPML1 . One method of 'chelating' PIPs is adding polycations such as polylysine to the cytoplasmic side of the membrane, where they bind the negatively charged phosphate head groups of PIPs in an electrostatic manner [26] , [27] . Polylysine at 500 μg ml −1 rapidly inhibited post-PI(3,5)P 2 I TRPML1 , but not I TRPML1-Va ( Fig. 3a–c ), indicating that polylysine primarily affected TRPML1 (activation) gating. In support, a neutralizing anti-PI(3,5)P 2 antibody at 5 μg ml −1 significantly inhibited post-PI(3,5)P 2 I TRPML1 , but not I TRPML1-Va ( Fig. 3d–f ). In contrast, no significant inhibition was seen with an anti-PI(4,5)P 2 antibody ( Fig. 3d,e ). To further investigate whether the basal I TRPML1 before PI(3,5)P 2 treatment was caused by basal levels of PI(3,5)P 2 in the endolysosomal membrane, we investigated a subset of vacuoles with large basal currents of >100 pA at −140 mV. Strong inhibitions were observed with polylysine (92±1%, N =7) or anti-PI(3,5)P 2 antibody (94±1%, N =10), but not with anti-PI(4,5)P 2 antibody (3±1%, N =4; Fig. 3g–i ). 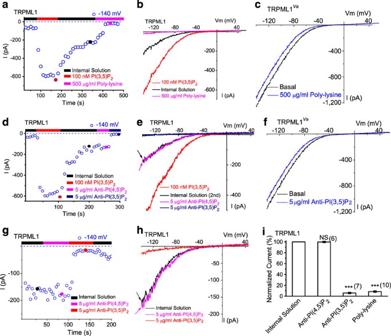Figure 3: A decrease in PI(3,5)P2by chelating agents suppresses TRPML1 channel activity in the endolysosomal membrane. (a) Post- PI(3,5)P2quasi-steady stateITRPML1was inhibited by bath (internal/cytoplasmic) application of poly-lysine (500 μg ml−1) to an enlarged endolysosome from a TRPML1-EGFP-expressing Cos-1 cell.ITRPML1increased with addition of 100 nM PI(3,5)P2, but gradually reduced to a quasi-steady state level upon washout. (b) Representative traces ofITRPML1at three time points, as shown ina: upon PI(3,5)P2application (red), washout (black), and poly-lysine application (magenta). (c) Lack of poly-lysine (500 μg ml−1) effect on whole-endolysosomeITRPML1-Va. (d) Post-PI(3,5)P2quasi-steady stateITRPML1was inhibited by bath application of neutralizing anti-PI(3,5)P2(5 μg ml−1), but not anti-PI(4,5)P2(5 μg ml−1). (e) Representative traces ofITRPML1at three time points, as shown ind. (f) Lack of anti-PI(3,5)P2(5 μg ml−1) effect on whole-endolysosomeITRPML1-Va. (g,h) Large basal pre-PI(3,5)P2ITRPML1was inhibited by bath application of neutralizing anti-PI(3,5)P2(5 μg ml−1), but not anti-PI(4,5)P2. (i)ITRPML1was inhibited by more than 90% by bath (internal/cytoplasmic) application of poly-lysine (500 μg ml−1) or PI(3,5)P2antibody. Data are presented as the mean±s.e.m.; thennumbers are in parentheses. Statistical comparisons were made using analysis of variance: ***P<0.001. Figure 3: A decrease in PI(3,5)P 2 by chelating agents suppresses TRPML1 channel activity in the endolysosomal membrane. ( a ) Post- PI(3,5)P 2 quasi-steady state I TRPML1 was inhibited by bath (internal/cytoplasmic) application of poly-lysine (500 μg ml −1 ) to an enlarged endolysosome from a TRPML1-EGFP-expressing Cos-1 cell. I TRPML1 increased with addition of 100 nM PI(3,5)P 2 , but gradually reduced to a quasi-steady state level upon washout. ( b ) Representative traces of I TRPML1 at three time points, as shown in a : upon PI(3,5)P 2 application (red), washout (black), and poly-lysine application (magenta). ( c ) Lack of poly-lysine (500 μg ml −1 ) effect on whole-endolysosome I TRPML1-Va . ( d ) Post-PI(3,5)P 2 quasi-steady state I TRPML1 was inhibited by bath application of neutralizing anti-PI(3,5)P 2 (5 μg ml −1 ), but not anti-PI(4,5)P 2 (5 μg ml −1 ). ( e ) Representative traces of I TRPML1 at three time points, as shown in d . ( f ) Lack of anti-PI(3,5)P 2 (5 μg ml −1 ) effect on whole-endolysosome I TRPML1-Va . ( g , h ) Large basal pre-PI(3,5)P 2 I TRPML1 was inhibited by bath application of neutralizing anti-PI(3,5)P 2 (5 μg ml −1 ), but not anti-PI(4,5)P 2 . ( i ) I TRPML1 was inhibited by more than 90% by bath (internal/cytoplasmic) application of poly-lysine (500 μg ml −1 ) or PI(3,5)P 2 antibody. Data are presented as the mean±s.e.m. ; the n numbers are in parentheses. Statistical comparisons were made using analysis of variance: *** P <0.001. Full size image To further confirm that PI(3,5)P 2 is an endogenous activator of TRPML1, we also recorded basal I TRPML1 after depleting the PI(3,5)P 2 level by overexpressing MTM1, a PI 3 phosphatase that can convert PI(3,5)P 2 and PI(3)P into PI(5)P and PI, respectively [11] , [15] . A rapamycin-dependent heterodimerization system was used to recruit the otherwise cytosolic MTM1 [28] (see Fig. 4a,b ). In cells expressing both RFP-FRB-MTM1 and EGFP-2*FKBP-Rab7, rapamycin induced a rapid recruitment of MTM1 to Rab7-positive LEL membranes ( Fig. 4b ). We noticed that basal I TRPML1 was consistently larger for vacuoles isolated from Cos-1 cells with longer (>5 h) pretreatment of vacuolin-1 (data not shown). In vacuoles isolated from MTM1-transfected cells, large basal I TRPML1 was observed before rapamycin treatment ( Fig. 4c ). However, after recruitment of MTM1 ( Fig. 4d ), but not the inactive mutant (C375S) MTM1 ( Fig. 4e ), a large suppression of basal whole-endolysosome I TRPML1 was seen ( Fig. 4d–f ). Collectively, these results suggest that PI(3,5)P 2 levels were the primary determinant of TRPML1 channel activity in the endolysosome. 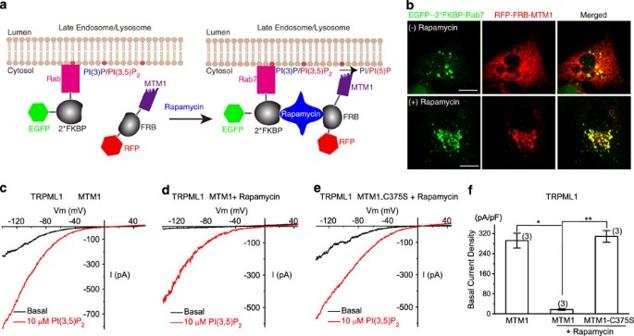Figure 4: A decrease in PI(3,5)P2level by a translocatable lipid phosphatase suppresses TRPML1 channel activity in the endolysosomal membrane. (a) Recruitment of MTM1 to endolysosomal membranes by rapamycin-dependent heterodimerization of RFP-FRB-MTM1 and EGFP-2*FKBP-Rab7. Rab7 is a LEL-specific Rab protein. MTM1 is a PI 3 phosphatase that can convert PI(3,5)P2and PI(3)P into PI(5)P and PI, respectively. (b) Rapamycin-dependent heterodimerization of RFP-FRB-MTM1 and EGFP-2*FKBP-Rab7 alters subcellular localization of MTM1. Cos-1 cells were transfected with both RFP-FRB-MTM1 and EGFP-2*FKBP-Rab7. Rapamycin (500 nM; 20 min) treatment promotes co-localization of MTM1-RFP with Rab7-EGFP. Scale Bar=10 μm. (c–f) The effects of MTM1 onITRPML1. Cos-1 cells were co-transfected with human TRPML1-myc, RFP-FRB-MTM1 or RFP-FRB-MTM1-C375S, and EGFP-2*FKBP-Rab7. MTM1 was recruited to LEL membranes by rapamycin (500 nM)-dependent heterodimerization of RFP-FRB-MTM1 and EGFP-2*FKBP-Rab7. (c)ITRPML1in MTM1-transfected cells before rapamycin treatment. (d)ITRPML1in MTM1-transfected cells after rapamycin treatment. (e)ITRPML1in MTM1-C357S-transfected cells after rapamycin treatment. (f) Differential effects of WT and inactive mutant (C375S) MTM1 on basal whole-endolysosomeITRPML1. Data are presented as the mean±s.e.m.; thennumbers are in parentheses. Statistical comparisons were made using analysis of variance: *P<0.05; **P<0.01. Figure 4: A decrease in PI(3,5)P 2 level by a translocatable lipid phosphatase suppresses TRPML1 channel activity in the endolysosomal membrane. ( a ) Recruitment of MTM1 to endolysosomal membranes by rapamycin-dependent heterodimerization of RFP-FRB-MTM1 and EGFP-2*FKBP-Rab7. Rab7 is a LEL-specific Rab protein. MTM1 is a PI 3 phosphatase that can convert PI(3,5)P 2 and PI(3)P into PI(5)P and PI, respectively. ( b ) Rapamycin-dependent heterodimerization of RFP-FRB-MTM1 and EGFP-2*FKBP-Rab7 alters subcellular localization of MTM1. Cos-1 cells were transfected with both RFP-FRB-MTM1 and EGFP-2*FKBP-Rab7. Rapamycin (500 nM; 20 min) treatment promotes co-localization of MTM1-RFP with Rab7-EGFP. Scale Bar=10 μm. ( c – f ) The effects of MTM1 on I TRPML1 . Cos-1 cells were co-transfected with human TRPML1-myc, RFP-FRB-MTM1 or RFP-FRB-MTM1-C375S, and EGFP-2*FKBP-Rab7. MTM1 was recruited to LEL membranes by rapamycin (500 nM)-dependent heterodimerization of RFP-FRB-MTM1 and EGFP-2*FKBP-Rab7. ( c ) I TRPML1 in MTM1-transfected cells before rapamycin treatment. ( d ) I TRPML1 in MTM1-transfected cells after rapamycin treatment. ( e ) I TRPML1 in MTM1-C357S-transfected cells after rapamycin treatment. ( f ) Differential effects of WT and inactive mutant (C375S) MTM1 on basal whole-endolysosome I TRPML1 . Data are presented as the mean±s.e.m. ; the n numbers are in parentheses. Statistical comparisons were made using analysis of variance: * P <0.05; ** P <0.01. Full size image Binding of PI(3,5)P 2 to the N terminus of TRPML1 in vitro Phosphoinoitides are known to bind with high affinity to PI-binding modules such as PH or FYVE domain, or to a poly-basic region with unstructured clusters of positively charged amino-acid residues, such as Arg and Lys, in an electrostatic manner [27] . PI(4,5)P 2 can bind directly to the cytoplasmic N- and C-termini of several plasma membrane TRPs [26] , [29] . Notably, the intracellular N terminus of TRPML1 has a poly-basic region [26] (see Fig. 5a ). To test whether PI(3,5)P 2 binds directly to TRPML1, we fused glutathione S -transferase (GST) to the entire N terminus of mouse TRPML1, up to residue 69 (see Fig. 5a for putative membrane topology). The protein, GST-TRPML1-N (abbreviated as GST-ML1-N), was used to probe PIPs immobilized on nitrocellulose membranes [26] , [27] , [29] . GST-ML1-N, but not GST alone, bound to PIP 3 and PIP 2 s, but not to other PIPs or phospholipids ( Fig. 5b ). A liposome assay showed that GST-ML1-N strongly associated with PI(3,5)P 2 , but not with PI(3)P or control liposomes ( Fig. 5c ). In a pull-down assay, agarose beads that conjugated with PI(3,5)P 2 , but not with control lipids, pulled down GST-ML1-N ( Fig. 5d ). Taken together, these results suggest that PI(3,5)P 2 bound directly in vitro to the cytoplasmic N terminus of TRPML1. 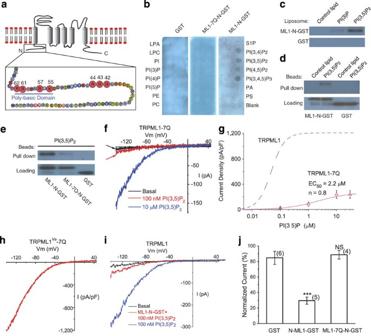Figure 5: Direct binding of PI(3,5)P2to the TRPML1 N terminus requires multiple positively charged amino-acid residues. (a) The cytoplasmic N terminus of TRPML1 contains a poly-basic region and clusters of positively charged amino-acid residues as potential PI(3,5)P2-binding sites. The positively charged amino-acid residues (Arg and Lys) that were mutated into neutral amino acids Gln (Q) in this study are shown with enlarged circles and their amino-acid residue numbers. (b) Protein-lipid overlays. The strip contained 15 different types of lipids. PA, phosphatidic acid; S1P, sphingosine-1-phosphate. Three purified proteins were used to probe the strip: GST alone (left panel), GST-fused to the N-terminal fragment of TRPML1 (ML1-N-GST; right panel), and Gln-substituted mutant of ML1-N-GST (ML1-7Q-N-GST; middle). Proteins were detected with anti-GST antibodies. (c) Liposome pull-down assay. Liposomes were incubated with purified GST-fusion proteins, centrifuged and associated proteins visualized by western blot with GST antibodies. (d) Binding of GST-ML1-N to agarose beads conjugated to PI(3,5)P2, but not control lipids; GST alone failed to pull down PI(3,5)P2-conjugated beads. (e) Compared with GST-ML1-N, GST-ML1-7Q-N exhibited significantly weaker binding to PI(3,5)P2-conjugated agarose beads. (f) Whole-endolysosomeITRPML1-7Qwas weakly activated by high concentrations of PI(3,5)P2. (g) PI(3,5)P2dose dependence ofITRPML1-7Q. Dotted line indicates the dose dependence ofITRPML1(replotted fromFig. 1d). (h) Large basal whole-endolysosomeITRPML1-Va-7Q. Charge-removing Gln substitutions (7Q) were introduced into the gain-of-functionVabackground. (i) GST-ML1-N peptide (5 μg ml−1) reduced PI(3,5)P2-dependent activation of whole-endolysosomeITRPML1. (j) Charge-removing Gln-substituted substitutions (7Q) abolished the inhibitory effect of GST-ML1-N peptide. Data are presented as the mean ± s.e.m.; thennumbers are in parentheses. Statistical comparisons were made using analysis of variance: ***P<0.001. Figure 5: Direct binding of PI(3,5)P 2 to the TRPML1 N terminus requires multiple positively charged amino-acid residues. ( a ) The cytoplasmic N terminus of TRPML1 contains a poly-basic region and clusters of positively charged amino-acid residues as potential PI(3,5)P 2 -binding sites. The positively charged amino-acid residues (Arg and Lys) that were mutated into neutral amino acids Gln (Q) in this study are shown with enlarged circles and their amino-acid residue numbers. ( b ) Protein-lipid overlays. The strip contained 15 different types of lipids. PA, phosphatidic acid; S1P, sphingosine-1-phosphate. Three purified proteins were used to probe the strip: GST alone (left panel), GST-fused to the N-terminal fragment of TRPML1 (ML1-N-GST; right panel), and Gln-substituted mutant of ML1-N-GST (ML1-7Q-N-GST; middle). Proteins were detected with anti-GST antibodies. ( c ) Liposome pull-down assay. Liposomes were incubated with purified GST-fusion proteins, centrifuged and associated proteins visualized by western blot with GST antibodies. ( d ) Binding of GST-ML1-N to agarose beads conjugated to PI(3,5)P 2 , but not control lipids; GST alone failed to pull down PI(3,5)P 2 -conjugated beads. ( e ) Compared with GST-ML1-N, GST-ML1-7Q-N exhibited significantly weaker binding to PI(3,5)P 2 -conjugated agarose beads. ( f ) Whole-endolysosome I TRPML1-7Q was weakly activated by high concentrations of PI(3,5)P 2 . ( g ) PI(3,5)P 2 dose dependence of I TRPML1-7Q . Dotted line indicates the dose dependence of I TRPML1 (replotted from Fig. 1d ). ( h ) Large basal whole-endolysosome I TRPML1-Va-7Q . Charge-removing Gln substitutions (7Q) were introduced into the gain-of-function Va background. ( i ) GST-ML1-N peptide (5 μg ml −1 ) reduced PI(3,5)P 2 -dependent activation of whole-endolysosome I TRPML1 . ( j ) Charge-removing Gln-substituted substitutions (7Q) abolished the inhibitory effect of GST-ML1-N peptide. Data are presented as the mean ± s.e.m. ; the n numbers are in parentheses. Statistical comparisons were made using analysis of variance: *** P <0.001. Full size image Critical amino-acid residues in PI(3,5)P 2 binding To further map the PI(3,5)P 2 -binding sites, we systematically replaced positively charged amino-acid residues (Arg and Lys) within and adjacent to the poly-basic region with non-charged Gln residues and assayed Gln-substituted, purified GST fusion proteins for PI(3,5)P 2 binding. We also tested whether PI(3,5)P 2 activated Gln-substituted TRPML1 channels using whole-endolysosome recordings. A dramatic decrease in PI(3,5)P 2 binding and activation ( Fig. 5e–g ) was observed in a 7Q mutant, with seven substitutions (R42Q/R43Q/R44Q/K55Q/R57Q/R61Q/K62Q; Fig. 5a ). In contrast to GST-ML1-N, GST-ML1-7Q-N failed to bind significantly to PI(3,5)P 2 or to other PIPs in the PIP strip and pull-down assays ( Fig. 5b,e ). Considering the specificity of PI(3,5)P 2 for TRPML1 activation, one plausible explanation for the apparent discrepancy between our biochemical assays (see Fig. 5b ) and electrophysiological measurements (see Fig. 1f ) is that the purified GST-ML1-N protein fragment did not recapitulate the specificity of PIP binding of full-length TRPML1 in the endolysosomal membrane. Nevertheless, the binding affinity of ML1-N to PI(3,5)P 2 was dramatically reduced by removing the charges with the 7Q mutations ( Fig. 5e ), suggesting that multiple positively charged amino-acid residues are critical for PI(3,5)P 2 binding. Compared with WT TRPML1, TRPML1-7Q was only weakly activated by high concentrations of PI(3,5)P 2 , with a maximal response (efficacy) that was approximately 20% of I TRPML1 (EC 50 =2.2±2 μM, Hill slope ( n )=0.8, N =6 vacuoles) ( Fig. 5f,g ). Similar to TRPML1 Va , TRPML1 Va -7Q also exhibited large basal currents ( Fig. 5h ), suggesting a relatively specific effect of 7Q mutations on PI(3,5)P 2 -dependent activation. Consistent with the PI(3,5)P 2 -binding assay results, we found that GST-ML1-N, but not GST-ML1-7Q-N, competitively reduced the activation effect of PI(3,5)P 2 ( Fig. 5i,j ). Collectively, our results suggest that PI(3,5)P 2 bound directly to the cytoplasmic N terminus of TRPML1, resulting in conformational changes that favour the opening of TRPML1. PI(3,5)P 2 in vacuolar Ca 2+ release in yeast TRPML1 is a Ca 2+ -permeable channel [30] , [31] ; hence activation by PI(3,5)P 2 may lead to Ca 2+ release from endolysosomes. Although PIKfyve/Fab1 is a PI 5 kinase that is responsible for PI(3,5)P 2 generation in both yeast and mammalian cells [11] , [13] , [14] , [15] , the extracellular signals that lead to activation of PIKfyve in mammalian cells have not been identified. Furthermore, endolysosomal Ca 2+ release has been difficult to detect in mammalian cells because of the small size of the endolysosome [5] , [32] . In contrast, Fab1-mediated PI(3,5)P 2 production has been well documented in yeast [11] , [13] . For example, hyperosmotic shock increases PI(3,5)P 2 levels more than 20-fold within a few minutes [11] , [13] . Interestingly, hyperosmotic shock is also known to induce Ca 2+ release from yeast vacuoles, which share many similar features with mammalian lysosomes. Induction of Ca 2+ release is through Yvc1/TRPY1, a TRP channel homologue in yeast, and occurs with a slightly faster, but otherwise comparable time course of PI(3,5)P 2 elevation [33] . On the basis of our data, we hypothesized that hyperosmolarity-induced vacuolar Ca 2+ release would be dependent on elevated PI(3,5)P 2 levels. To test this, we used a luminescence assay based on aequorin, a genetic Ca 2+ sensor [33] , to measure changes in cytosolic Ca 2+ ([Ca 2+ ] cyt ) levels. Consistent with previous reports [33] , hyperosmotic shock by addition of 0.9 M NaCl to the culture medium induced a rapid and dramatic increase of [Ca 2+ ] cyt . The time required for peak [Ca 2+ ] cyt increase was 48±4 s, ( N =10 yeast colonies per experiments); the increase in luminescence was 700±94% over basal ( N =4; Fig. 6a,b ). In the yvc1 Δ mutant, however, no significant increase in [Ca 2+ ] cyt was observed (29±6% over basal, N =4), consistent with the hypothesis that the [Ca 2+ ] cyt increase resulted primarily from vacuolar release through Yvc1 [33] . Interestingly, in the fab1 Δ mutant, hyperosmotic shock also failed to induce any significant increase in [Ca 2+ ] cyt (20±8%, N =4; Fig. 6a,b ), in comparison with 700% for WT cells. Both yvc1 Δ and fab1 Δ cells responded to 14% ethanol or 0.03% SDS (data not shown), which is known to induce Ca 2+ influx [33] . Consistent with previous studies [11] , [13] , fab1 Δ mutant yeasts failed to exhibit vacuolar fragmentation in response to hyperosmotic shock ( Fig. 6c ). 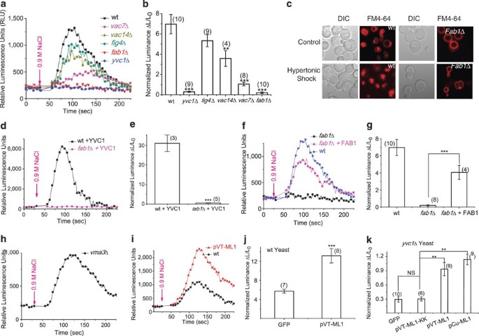Figure 6: Ca2+release from yeast vacuoles after hyperosmostic shock is dependent on PI(3,5)P2production. (a) Representative Ca2+response measured with aequorin-mediated luminescence in wild-type (WT),yvc1Δ, and PI(3, 5P)2-deficient strains (vac7Δ,vac14Δ,fig4Δ,fab1Δ) upon hyperosmotic shock induced by addition of 0.9 M NaCl. (b) Quantitative data to show luminescence responses upon hyperosmotic shock in different yeast strains. Fold-response was normalized to basal luminescence before shock. (c) Hyperosmotic shock increases the number of vacuoles and decreases the vacuolar volume in WT, but not fab1 mutant yeast strains. Both WT andfab1Δ cells were labelled with FM4-64 dye to visualize vacuole volume and the number of vacuole lobes. Cells were treated with 0.45 M NaCl and viewed by fluorescence microscopy. (d,e) Overexpression of YVC1 infab1Δ cells failed to restore hyperosmolarity-induced Ca2+response. (f,g) Overexpression ofFAB1infab1Δ cells restored hyperosmolarity-induced Ca2+response. (h,i) Overexpression of TRPML1 in WT yeast cells increased hyperosmolarity-induced Ca2+response. (j) Hyperosmotic shock induces vacuolar Ca2+release invma3mutant yeast strains. (k) Overexpression of TRPML1, but not pore mutant TRPML1-KK (in pCu and pVT expression vectors), inyvc1Δ yeast cells resulted in a small but significant hyperosmolarity-induced Ca2+response. Data ine,g,j,kare presented as the mean ± s.e.m.; thennumbers are in parentheses. Statistical comparisons were made using analysis of variance: **P<0.01; ***P<0.001. Figure 6: Ca 2+ release from yeast vacuoles after hyperosmostic shock is dependent on PI(3,5)P 2 production. ( a ) Representative Ca 2+ response measured with aequorin-mediated luminescence in wild-type (WT), yvc1 Δ, and PI(3, 5P) 2 -deficient strains ( vac7 Δ, vac14 Δ, fig4 Δ, fab1 Δ) upon hyperosmotic shock induced by addition of 0.9 M NaCl. ( b ) Quantitative data to show luminescence responses upon hyperosmotic shock in different yeast strains. Fold-response was normalized to basal luminescence before shock. ( c ) Hyperosmotic shock increases the number of vacuoles and decreases the vacuolar volume in WT, but not fab1 mutant yeast strains. Both WT and fab1 Δ cells were labelled with FM4-64 dye to visualize vacuole volume and the number of vacuole lobes. Cells were treated with 0.45 M NaCl and viewed by fluorescence microscopy. ( d , e ) Overexpression of YVC1 in fab1 Δ cells failed to restore hyperosmolarity-induced Ca 2+ response. ( f , g ) Overexpression of FAB1 in fab1 Δ cells restored hyperosmolarity-induced Ca 2+ response. ( h , i ) Overexpression of TRPML1 in WT yeast cells increased hyperosmolarity-induced Ca 2+ response. ( j ) Hyperosmotic shock induces vacuolar Ca 2+ release in vma3 mutant yeast strains. ( k ) Overexpression of TRPML1, but not pore mutant TRPML1-KK (in pCu and pVT expression vectors), in yvc1 Δ yeast cells resulted in a small but significant hyperosmolarity-induced Ca 2+ response. Data in e , g , j , k are presented as the mean ± s.e.m. ; the n numbers are in parentheses. Statistical comparisons were made using analysis of variance: ** P <0.01; *** P <0.001. Full size image Fab1 kinase activity is regulated by Vac7, Vac14 and Fig4, mutations with a partial or nearly complete loss of Fab1-mediated PI(3,5)P 2 production [11] , [12] , [13] , [15] , [34] . All these mutants exhibited reduced vacuolar Ca 2+ release: 533±60% ( N =4) for fig4 Δ; 357±77% ( N =4) for vac14 Δ; and 106±18% ( N =4) for vac7 Δ ( Fig. 6a,b ). The degree of Ca 2+ release reduction ( fab1 Δ> vac7 Δ> vac14 Δ> fig4 Δ) correlated well with the severity of the defect of PI(3,5)P 2 production in these strains [11] . The loss of Ca 2+ response in fab1 Δ cells was not due to reduced expression of Yvc1 ( Fig. 6d,e ), as transformation of Yvc1-GFP failed to restore the response. In contrast, when WT yeast FAB1 was transformed into fab1 Δ mutant yeast, hyperosmolarity-induced [Ca 2+ ] cyt increase was largely restored ( Fig. 6f,g ). Mutant fab1 Δ yeasts reportedly hypoacidify the vacuole [11] , [13] , which could result in reduced Ca 2+ release because of a decrease in H + -dependent refilling of vacuolar Ca 2+ stores mediated by Vcx1 (vacuolar Ca 2+ -H + exchanger) [35] . However, vcx1 Δ cells exhibit normal Ca 2+ release in response to hyperosmotic shock [33] , indicating that the alternate Pmc1 (vacuolar Ca 2+ ATPase)-mediated refilling system is sufficient to maintain vacuolar Ca 2+ stores. In support, we found that hypoacidified cells lacking vma3 , an essential component of vacuolar ATPase [35] , exhibited normal [Ca 2+ ] cyt release ( Fig. 6h ). These results suggested that the Fab1-mediated PI(3,5)P 2 generation system was required for hyperosmolarity-induced, Yvc1-dependent vacuolar Ca 2+ release. Although TRPML1 shares a degree of sequence homology to Yvc1, they differ significantly in their channel properties [5] , [36] . To test whether TRPML1 functions in yeast, we overexpressed TRPML1 in both a WT and yvc1 Δ background. Overexpression of TRPML1 in WT yeast resulted in a significant increase in Ca 2+ release in response to hyperosmotic shock ( Fig. 6i,j ). In yvc1 Δ cells, overexpression of TRPML1, but not a non-functional pore mutant of TRPML1 (TRPML1-KK), resulted in a partial rescue of the [Ca 2+ ] cyt response, with a 114±14% increase over basal luminescence ( N =9) ( Fig. 6k ). In contrast, overexpression of TRPML1 in fab1 Δ failed to result in significant [Ca 2+ ] cyt response ( Supplementary Fig. S5 ), whereas overexpression of YVC1 in yvc1 Δ cells completely restored the [Ca 2+ ] cyt response ( Supplementary Fig. S6 ). The rescue might be incomplete because Yvc1, but not TRPML1, is activated by cytoplasmic Ca 2+ and mechanical force [36] , both of which might have synergistic effects with PI(3,5)P 2 . Nevertheless, these results suggest that regulation of lysosomal Ca 2+ channels by PI(3,5)P 2 might be a conserved mechanism in eukaryotic cells. TRPML1 and PI(3,5)P 2 in endolysosomal trafficking The data presented here suggest that TRPMLs might be activated downstream of the PI(3,5)P 2 increase to trigger membrane fusion and fission (see Supplementary Fig. S1 ). If this hypothesis is correct, expression of TRPML1, which often exhibits substantial basal activity in heterologous systems [5] , might alleviate trafficking defects in PI(3,5)P 2 -deficient cells. In cultured Vac14 −/− fibroblast cells, the trafficking defects from PI(3,5)P 2 deficiency were reflected by enlarged vacuoles/LELs (>3 up to 12 μm in diameter) in 79±7% of cells ( N =3 experiments with >100 cells) ( Fig. 7a ; study by Zhang et al . [12] ). Only approximately 5–10% of WT cells were vacuolated (<4 μm; data not shown). Transfection of a WT Vac14 construct was sufficient to restrict vacuoles to 15±2% of cells ( N =3 experiments; Fig. 7a ). Interestingly, we were able to rescue the vacuolar phenotype by transfection of TRPML1, which showed vacuolation in 18±1% cells ( N =6), but not pore-mutant TRPML1 (ML1-KK) with 69±6% vacuolation ( N =3), or the PI(3,5)P 2 -insensitive mutant TRPML1 (ML1-7Q) with 75±7% vacuolation ( N =3) ( Fig. 7a–d ). Although ML1-7Q still localized to Lamp1-positive compartments ( Fig. 7b,e ), large vacuoles were seen in the majority of ML1-7Q-transfected Vac14 −/− fibroblasts ( Fig. 7a–d ). Collectively, these results suggested that TRPML1 channel activity and PI(3,5)P 2 sensitivity had important roles in controlling vacuole size. 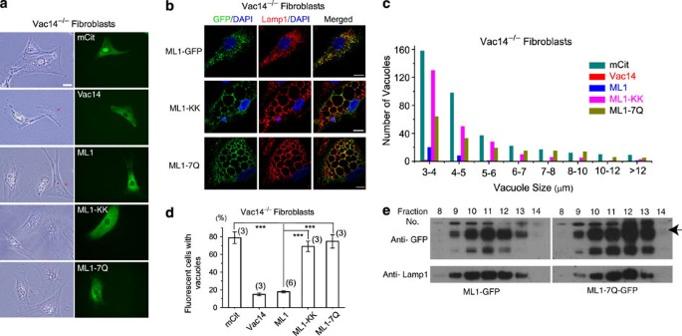Figure 7: Overexpression of TRPML1 rescues the enlarged endolysosome phenotype of PI(3,5)P2-deficient mouse fibroblasts. (a,b) The effects of overexpression of WT TRPML1 and pore (ML1-KK) or PI(3,5)P2-insensitive (ML1-7Q) mutant TRPML1 on the number and size of the vacuoles in Vac14−/−fibroblasts. Cultured Vac14−/−mouse fibroblast cells exhibited variable numbers (1–20) of large (>3 μm) vacuoles/endolysosomes. Left, differential interference contrast image, right epifluorescence. Green fluorescence, mCit (vector only), mCit-Vac14, GFP-ML1, GFP-ML1-KK, GFP-ML1-7Q. Non-vacuolated cells are indicated by asterisk. Scale bar, 20 μm. (b) TRPML1, ML1-KK and ML1-7Q proteins were co-localized in Lamp1-positive compartments of Vac14−/−fibroblast cells. (c) Histogram analysis of the vacuole size/number in Vac14−/−fibroblasts transfected with indicated constructs. (d) Large vacuoles in 75% of vector (mCit)-transfected Vac14−/−fibroblast cells. Overexpression of Vac14-mCit or EGFP-ML1 reduced the percentage (of enlarged vacuoles) to approximately 15%, whereas the 75% of EGFP-ML1-KK or EGFP-ML1-7Q-transfected cells contained enlarged vacuoles. Data are presented as the mean ± s.e.m.; thennumbers are in parentheses. Statistical comparisons were made using analysis of variance: ***P<0.001. (e) Cellular organelle fractionation analysis reveals co-localization of TRPML1 and TRPML1-7Q with Lamp-1. Gradient cellular fractionations were obtained using ultracentrifugation. Both TRPML1 and TRPML1-7Q proteins were concentrated in Lamp1-rich fractionations. Arrow shows full-length TRPML1-EGFP. Figure 7: Overexpression of TRPML1 rescues the enlarged endolysosome phenotype of PI(3,5)P 2 -deficient mouse fibroblasts. ( a , b ) The effects of overexpression of WT TRPML1 and pore (ML1-KK) or PI(3,5)P 2 -insensitive (ML1-7Q) mutant TRPML1 on the number and size of the vacuoles in Vac14 −/− fibroblasts. Cultured Vac14 −/− mouse fibroblast cells exhibited variable numbers (1–20) of large (>3 μm) vacuoles/endolysosomes. Left, differential interference contrast image, right epifluorescence. Green fluorescence, mCit (vector only), mCit-Vac14, GFP-ML1, GFP-ML1-KK, GFP-ML1-7Q. Non-vacuolated cells are indicated by asterisk. Scale bar, 20 μm. ( b ) TRPML1, ML1-KK and ML1-7Q proteins were co-localized in Lamp1-positive compartments of Vac14 −/− fibroblast cells. ( c ) Histogram analysis of the vacuole size/number in Vac14 −/− fibroblasts transfected with indicated constructs. ( d ) Large vacuoles in 75% of vector (mCit)-transfected Vac14 −/− fibroblast cells. Overexpression of Vac14-mCit or EGFP-ML1 reduced the percentage (of enlarged vacuoles) to approximately 15%, whereas the 75% of EGFP-ML1-KK or EGFP-ML1-7Q-transfected cells contained enlarged vacuoles. Data are presented as the mean ± s.e.m. ; the n numbers are in parentheses. Statistical comparisons were made using analysis of variance: *** P <0.001. ( e ) Cellular organelle fractionation analysis reveals co-localization of TRPML1 and TRPML1-7Q with Lamp-1. Gradient cellular fractionations were obtained using ultracentrifugation. Both TRPML1 and TRPML1-7Q proteins were concentrated in Lamp1-rich fractionations. Arrow shows full-length TRPML1-EGFP. Full size image We used biochemical binding assays to demonstrate that PI(3,5)P 2 binds directly to the N terminus of TRPML1. Using whole-endolysosomal patch-clamp recordings, we showed that PI(3,5)P 2 robustly activates TRPML1 in the endolysosome. The effect of PI(3,5)P 2 was strikingly specific; none of the other PIPs activated TRPML1. Using a spectrum of yeast mutant strains with variable degrees of PI(3,5)P 2 deficiency, we established a high-degree of correlation between the amount of vacuolar Ca 2+ release and the levels of PI(3,5)P 2 . Finally, we showed that overexpression of WT, but not the PIP 2 -insensitive variant of TRPML1, was sufficient to rescue the trafficking defects in PI(3,5)P 2 -deficient mammalian cells, as demonstrated by observing enlarged vacuoles. Our identification of an endolysosome-localizing Ca 2+ channel that is activated by the endolysosome-specific PI(3,5)P 2 provides a previously unknown link between these two important regulators of intracellular membrane trafficking. Similar trafficking defects are seen in both TRPML1 −/− cells and PI(3,5)P 2 -deficient cells. For example, LEL-to-Golgi retrograde trafficking, a process requiring membrane fission, is defective in both TRPML1 −/− cells [5] , [19] , [37] , [38] , [39] and PI(3,5)P 2 -deficient cells [11] , [12] , [13] , [14] , [15] , [34] . Furthermore, both TRPML1 and PI(3,5)P 2 -metabolizing enzymes are implicated in membrane-fusion processes such as exocytosis [11] , [15] , [20] , and lysosomal fusion with autophagosomes [6] , [40] . Thus, both TRPML1 and PI(3,5)P 2 have active roles in membrane fission and fusion. However, the cellular defects of PI(3,5)P 2 -deficient cells are generally more severe than those of TRPML1 −/− cells. PI(3,5)P 2 is proposed to have at least five independent functions, including recruitment of cytosolic proteins to define organelle specificity; functional regulation of endolysosomal membrane proteins; determination of physical properties and fusogenic potential of endolysosomal membranes; and serving as a precursor for PI(3)P or PI(5)P, and modulating endolysomal pH [9] , [11] , [15] . Hence, activation of TRPML1 might define a subset of the multiple functions of PI(3,5)P 2 . Such activation, however, may provide an essential spatial and temporal regulation of endolysosomal dynamics. Membrane fusion and fission are highly coordinated processes requiring an array of cytosolic and membrane-bound proteins and factors. A local increase in PI(3,5)P 2 likely recruits protein complexes required to generate the membrane curvature necessary for membrane fusion and fission [15] . A local increase in PI(3,5)P 2 could also activate TRPML1 to elevate juxtaorganellar Ca 2+ , which binds to a putative Ca 2+ sensor protein such as Synaptotagmin/CaM [3] or ALG-2 [41] to exert effects on SNARE proteins or lipid bilayer fusion [15] , [42] . A similar mechanism might be used by NAADP and TPC channels to regulate membrane trafficking in the endolysosome [32] , [43] . The remarkable specificity of PI(3,5)P 2 in activating TRPML1 is consistent with the role of Ca 2+ in controlling the direction and specificity of membrane traffic [1] , [3] . Although we identified several positively charged amino-acid residues as potential PI(3,5)P 2 -binding sites, electrostatic interaction alone is unlikely to provide a high-affinity PI(3,5)P 2 -binding pocket [26] , [27] . Thus, additional structural determinants such as hydrophobic amino-acid residues must also contribute to specificity by interacting with the lipid portion of PI(3,5)P 2 . Because of the low abundance of PI(3,5)P 2 [11] , such specificity might be a prerequisite for PI(3,5)P 2 and TRPML1 to control the trafficking direction in the late endocytic pathway. In other organelles, however, other PIPs and intracellular Ca 2+ channels are likely to provide machinery necessary for Ca 2+ -dependent membrane fission and fusion. Within LELs, membrane fusion and fission are likely to occur in suborganellar compartments that are enriched for both TRPMLs and PIKfyve. Although TRPML-mediated juxtaorganellar Ca 2+ transients might be captured using real-time live-imaging methods, these seemingly 'spontaneous' events may correlate with membrane fusion and fission events that can be simultaneously monitored with fluorescence imaging approaches. Molecular biology and biochemistry Full-length mouse TRPML1, 2 and 3 were cloned into the EGFP-C2 (Clontech) or mCherry vector [20] , [21] , [31] . TRPML1 non-conducting pore mutant (D471K/D472K; abbreviated TRPML1-KK) and PIP 2 -insensitive mutant (R42Q/R43Q/R44Q/K55Q/R57Q/R61Q/K62Q; abbreviated TRPML1-7Q) were constructed using a site-directed mutagenesis kit (Qiagen). For GST fusion constructs, DNA fragments corresponding to the N-terminal (amino-acid residues 1–69) regions of mouse TRPML1 were generated by PCR amplification and cloned into the Eco RI and Xho I site of pGEX4T1 in frame to generate GST fusion protein plasmids (pGEX-ML1-N). For overexpression of TRPML1 in yeast, full-length mouse TRPML1 was cloned into the Xho I and Eco RI site of the pCuGFP416 vector, and the Xho I and Hin dIII site of the pVT102U-GFP vector. FKBP*2 fragment was PCR-amplified from EGFP-FKBP12-Rab5 and inserted into the Hin dIII and Xho I site of EGFP-Rab7 vector. RFP-FRB-MTM1 and EGFP-FKBP*2-Rab5 were kind gifts from Dr Banasfe Larijani. All constructs were confirmed by sequencing, and protein expression was verified by western blot. HEK293 T, Cos-1, human fibroblasts or mouse primary fibroblast cells were transiently transfected with TRPML1-3 and TRPML1 mutants for electrophysiology, biochemistry, live-cell imaging and confocal imaging. Confocal images were taken using a Leica (TCS SP5) microscope. TRPML1 western blot analyses were performed with an anti-GFP monoclonal antibody (Covance). Endolysosomal electrophysiology Endolysosomal electrophysiology was performed in isolated endolysosomes using a modified patch-clamp method [20] , [21] . HEK293 or Cos-1 cells were used for all the heterologous expression experiments and were transfected using Lipofectamine 2000 (Invitrogen) with TRPML1 or mutants fused to GFP or mCherry. Human skin fibroblast cells from an ML4 patient (TRPML1 −/− , clone GM02048) and age-matched control (TRPML1 +/+ , clone GM00969) were obtained from the Coriell Institute for Medical Research (NJ, USA). LEL size is usually <0.5 μm, which is suboptimal for patch clamping. We therefore treated cells with 1 μM vacuolin-1, a lipid-soluble polycyclic triazine that can selectively increase the size of endosomes and lysosomes, for ∼ 1 h [44] . Large vacuoles (up to 5 μm; capacitance=0.68±0.05 pF, N =44 vacuoles) were observed in most vacuolin-treated cells. Occasionally, enlarged LELs were obtained from TRPML1-transfected cells without vacuolin-1 treatment. No significant difference in TRPML channel properties was observed for enlarged LELs obtained with or without vacuolin-1 treatment. Vacuoles positive for both mCherry-TRPML1 and EGFP-Lamp1 were considered enlarged LELs. Whole-endolysosome recordings were performed on isolated enlarged LELs. In brief, a patch pipette (electrode) was pressed against a cell and quickly pulled away to slice the cell membrane. Enlarged LELs were released into a dish and identified by monitoring EGFP-TRPML1, the mCherry-TRPML1 or EGFP-Lamp1 fluorescence. Unless otherwise stated, bath (internal/cytoplasmic) solution contained 140 mM K-Gluconate, 4 mM NaCl, 1 mM EGTA, 2 mM Na 2 -ATP, 2 mM MgCl 2 , 0.39 mM CaCl 2 , 0.1 mM GTP and 10 mM HEPES (pH adjusted with KOH to 7.2; free [Ca 2+ ] i approximately 100 nM). The pipette (luminal) solution was pH 4.6 standard extracellular solution (modified Tyrode's) with 145 mM NaCl, 5 mM KCl, 2 mM CaCl 2 , 1 mM MgCl 2 , 20 mM HEPES and 10 mM glucose (pH adjusted with NaOH). All bath solutions were applied by means of a fast perfusion system to achieve a complete solution exchange within a few seconds. Data were collected using an Axopatch 2A patch clamp amplifier, Digidata 1440, and pClamp 10.0 software (Axon Instruments). Whole-endolysosome currents were digitized at 10 kHz and filtered at 2 kHz. All experiments were conducted at room temperature (21–23 °C), and all recordings were analysed using pCLAMP10 (Axon Instruments) and Origin 8.0 (OriginLab). All PIP antibodies are from Echelon Biosciences. All PIPs are from A.G. Scientific. GST fusion proteins To purify GST-tagged proteins, Escherchia coli BL21DE3 was transformed with empty pGEX vectors or with pGEX-TRPML1-N (abbreviated as pGEX-ML1-N). After growth to approximately OD 600 =0.6 in a SuperBroth medium supplemented with ampicillin, expression was induced with isopropylthiogalactoside (1 mM) for 7 h at 37 °C. Cells were collected and resuspended in 30 ml of ice-cold PBS supplemented with protease inhibitor cocktail, 0.5 mM EDTA and deoxytibonuclease, and lysed with a French press. Cell lysates in 1% Triton X-100 were incubated with 2 ml of mixed glutathione Sepharose (GE Healthcare) for 1 h at 4 °C. After three washes with 30 ml PBS, proteins were eluted with 7 ml elution buffer (10 mM Glutathione, 50 mM Tris, pH 8). Lipid strip-binding assay Lipid-binding analysis of GST-ML1-N and GST-ML1-7Q-N fusion proteins was conducted using PIP Strips (Echelon Biosciences), with each spot containing 100 pmol of active lipids. Membranes were blocked with PBS Tween (PBST) solution (supplemented with 3% fatty acid-free bovine serum albumin) for 1 h at room temperature, and incubated with 0.5–3 μg GST fusion protein in blocking buffer overnight. After six washes, the membranes were incubated with a mouse anti-GST antibody (1:5,000, Sigma) for 1 h at room temperature, and secondary antibody horseradish peroxidase-labelled goat anti-mouse (1:5,000) was added before detection by enhanced chemiluminescence. PIP bead-binding assay Purified GST fusion proteins (10 μg) were diluted in 1 ml of binding buffer (50 mM Tris, 150 mM NaCl, 0.25% NP-40, pH 7.5) and incubated with 50 μl of 50% lipid-conjugated Sepharose beads (Echelon Biosciences) for 2 h. After three washes, proteins were eluted from the PIP beads by heating at 50 °C for 10 min in 2× SDS-polyacrylamide gel electrophoresis sample buffer and visualization was performed by western blot. Liposome binding assay Purified GST fusion proteins (3 μg) were incubated with 20 μl liposome (Echelon Biosciences) in 1 ml of binding buffer (50 mM Tris, 150 mM NaCl, 0.05% Non-idet P-40, pH 7.5) for 10 min. Liposomes were pelleted at 16,000× g for 10 min and washed multiple times with binding buffer. Bound fractions were analysed by western blot. Yeast strains WT and mutant yeast strains are listed in Table 1 . Strains were grown at 24 or 30 °C in either YPD (yeast extract/peptone/glucose) or synthetic complete minimal medium. Table 1 Yeast strains. Full size table Yeast Ca 2+ imaging Yeast Ca 2+ imaging experiments were conducted using an aequorin-based genetic Ca 2+ sensor method [33] . PEVP11/AEQ plasmid was kindly provided by Dr Patrick H. Masson (University of Wisconsin-Madison, Madison, WI). Transformed yeasts were inoculated from a saturated overnight culture to OD 600 ∼ 0.3 in a synthetic defined (SD) medium with 3 μM coelenterazine, and grown overnight (OD 600 =2–3) at 24 or 30 °C to convert apo-aequorin to aequorin. For each experiment, an aliquot of 250 μl was collected, resuspended in 100 μl SD medium and transferred to 94-well plates for luminescence measurement. Baseline luminescence was recorded every 3 s for 30 s using a PHERAstar plate reader (BMG Labs). Hyperosmotic shock was performed by adding an equal volume of SD medium (100 μl) containing 1.8 M of NaCl to a final concentration of 0.9 M. All experiments were concluded with 14% ethanol or 0.03% SDS, which resulted in maximal luminescence and served as a positive control for aequorin transformation. Yeast vacuole labelling Log-phase yeast cells were labelled with FM4-64 dye (Molecular Probes) [34] . Phase contrast and fluorescence images were taken using a Zeiss microscope with a ×100 objective. Mouse fibroblast vacuole assay Vac14 −/− mouse fibroblast cells were isolated and cultured as described previously [12] . Briefly, fibroblasts were transiently transfected by electroporation (260 V, 950 μF) with 100 μg of the following expression constructs: mCit, mCit-Vac14, GFP-ML1, GFP-ML1-KK or GFP-ML1-7Q. Cells were grown on 100-mm plates to 90% confluence and distributed to six 35-mm plates after electroporation. Cells were fixed with 4% paraformaldehyde 24 h after electroporation. Fibroblasts were considered to be vacuolated if they had at least one enlarged (>3 μm) cytoplasmic vacuole. Cellular fractionation To perform lysosomal fractionation studies [45] , cell lysates were obtained by Dounce homogenization in a homogenizing buffer (0.25 M sucrose, 1 mM Na 2 EDTA, 10 mM HEPES, pH 7.0). Lysates were then centrifuged at 1,900 g at 4 °C for 10 min to remove nuclei and intact cells. Postnuclear supernatants underwent ultracentrifugation through a Percoll density gradient using a Beckman L8-70 ultracentrifuge. An ultracentrifuge tube was layered with 2.5 M sucrose, 18% Percoll in homogenizing buffer and the postnuclear supernatant on top. Centrifugation was 67,200 g at 4 °C for 1.5 h in a Beckman Coulter 70.1 Ti Rotor. Samples were fractionated into 16 samples of unequal volume. Top fractions contained minimal cellular components, bottom fractions contained concentrated bands of cellular organelles and were separated into smaller fraction volumes. Confocal imaging All images were obtained using a Leica (TCS SP5) confocal microscope. Lamp1 antibody was from the Iowa Hybridoma Bank. Data analysis Data are presented as the mean ± s.e.m. Statistical comparisons were made using analysis of variance. A P -value <0.05 was considered statistically significant.